X-ray structure of a CDP-alcohol phosphatidyltransferase membrane enzyme and insights into its catalytic mechanism Phospholipids have major roles in the structure and function of all cell membranes. Most integral membrane proteins from the large CDP-alcohol phosphatidyltransferase family are involved in phospholipid biosynthesis across the three domains of life. They share a conserved sequence pattern and catalyse the displacement of CMP from a CDP-alcohol by a second alcohol. Here we report the crystal structure of a bifunctional enzyme comprising a cytoplasmic nucleotidyltransferase domain (IPCT) fused with a membrane CDP-alcohol phosphotransferase domain (DIPPS) at 2.65 Å resolution. The bifunctional protein dimerizes through the DIPPS domains, each comprising six transmembrane α-helices. The active site cavity is hydrophilic and widely open to the cytoplasm with a magnesium ion surrounded by four highly conserved aspartate residues from helices TM2 and TM3. We show that magnesium is essential for the enzymatic activity and is involved in catalysis. Substrates docking is validated by mutagenesis studies, and a structure-based catalytic mechanism is proposed. Phospholipids are not only major structural components of biological membranes but they also have key roles in cell physiology, regulation and maturation of numerous cellular processes [1] . Disruption of phospholipid homeostasis is associated with several human diseases, and has a crucial role in pathogen invasion, infectivity and virulence [1] , [2] . A better understanding of their metabolic pathways and regulation should help development of chemotherapeutic drugs against cancer and various infectious diseases. As an example, the synthesis of phosphatidylinositol is essential for growth of Mycobacterium smegmatis [3] and differs from the human pathway [4] , highlighting the respective biosynthetic enzymes as promising targets for the development of drugs to treat tuberculosis, the second cause of mortality by infectious diseases. To shed light into de novo biosynthesis of phospholipids, we characterized the structure of a representative from the CDP-alcohol phosphatidyltransferase family (CDP-OH_P_trans). Kennedy et al. [5] , [6] first described these enzymes using both an insoluble substrate (diacylglycerol) and a soluble substrate (CDP-alcohol). To date, more than 12,750 sequences are classified as CDP-OH_P_trans in UniProt Knowledgebase. Members of this family are integral membrane proteins that share a conserved sequence pattern and usually comprise 150–400 amino-acid residues. They catalyse the displacement of CMP from a CDP-alcohol by a second alcohol with formation of a phosphodiester bond and concomitant breaking of a phosphoride anhydride bond, having a key role in the biosynthesis of essential phospholipids. 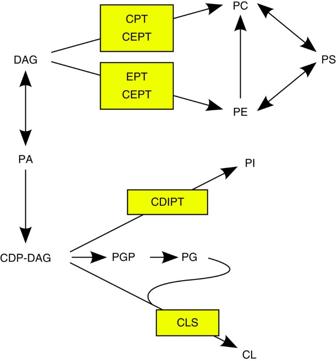Figure 1: Pathways of (glycero)phospholipid biosynthesis in mammalian cells. The biosynthesis starts either from diacylglycerol (DAG) or phosphatidic acid (PA), and results in production of phosphatidylcholine (PC), phosphatidyletanolamine (PE), phosphatidylserine (PS), phosphatidylinositol (PI) and cardiolipin (CL), adapted from Hermanssonet al.7The intermediate metabolites are CDP-DAG, phosphatidylglycerol phosphate (PGP) and phosphatidylglycerol (PG). The CDP-alcohol phosphatidyltransferase family enzymes in human are highlighted; CPT, cholinephosphotransferase 1; CEPT, choline/ethanolaminephosphotransferase 1; EPT, ethanolaminephosphotransferase 1; CDIPT, phosphatidylinositol synthase 1; and CLS, cardiolipin synthase. Figure 1 illustrates the participation of these enzymes in the biosynthesis of all major (glycero)phospholipids in mammalian cells [7] , including human phosphatidylinositol synthase, choline/ethanolaminephosphotransferase and cardiolipin synthase. Despite the important function of CDP-alcohol phosphotransferases, no structure had been yet characterized for any member. Figure 1: Pathways of (glycero)phospholipid biosynthesis in mammalian cells. The biosynthesis starts either from diacylglycerol (DAG) or phosphatidic acid (PA), and results in production of phosphatidylcholine (PC), phosphatidyletanolamine (PE), phosphatidylserine (PS), phosphatidylinositol (PI) and cardiolipin (CL), adapted from Hermansson et al. [7] The intermediate metabolites are CDP-DAG, phosphatidylglycerol phosphate (PGP) and phosphatidylglycerol (PG). The CDP-alcohol phosphatidyltransferase family enzymes in human are highlighted; CPT, cholinephosphotransferase 1; CEPT, choline/ethanolaminephosphotransferase 1; EPT, ethanolaminephosphotransferase 1; CDIPT, phosphatidylinositol synthase 1; and CLS, cardiolipin synthase. Full size image Since very often membrane proteins, especially those from human sources, resist crystallization we selected an enzyme from the hyperthermophilic archaeon Archaeoglobus fulgidus , which comprises CTP:L- myo -inositol-1-phosphate cytidylyltransferase (IPCT) fused with CDP-L- myo -inositol: myo -inositolphosphotransferase, also designated di- myo -inositol-1,3′-phosphate-1′-phosphate synthase (DIPPS), a member of the CDP-alcohol phosphatidyltransferase family. The bifunctional enzyme IPCT/DIPPS catalyses two consecutive steps of di- myo -inositol-1,3′-phosphate (DIP) biosynthesis [8] , [9] , [10] ( Fig. 2 ). For sake of simplicity ‘L’ and ‘ myo ’ will be omitted hereafter. First, inositol-1-phosphate is activated to CDP-inositol by IPCT. CMP is then displaced from CDP-inositol by inositol-1-phosphate with formation of DIP-phosphate (DIPP) by DIPPS. Finally, DIPP is dephosphorylated to DIP by a DIPP-phosphatase. DIP content increases drastically at supraoptimal growth temperatures and was shown to stabilize proteins in vitro [8] , [11] . Accordingly, DIP was proposed to be a major protecting molecule in a number of (hyper)thermophilic species of archaea and bacteria. In most organisms, both the IPCT and DIPPS activities are present in a single gene product, but separate genes can also be found [8] , [12] . 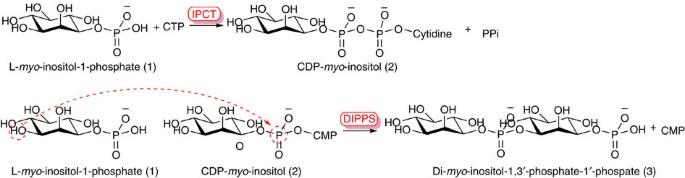Figure 2: Catalytic reactions of IPCT/DIPPS bifunctional enzyme. Biosynthesis of di-myo-inositol-1,3′-phosphate-1′-phosphate (DIPP). IPCT-CTP:L-myo-inositol-1-phosphate cytidylyltransferase; DIPPS-CDP-L-myo-inositol:myo-inositolphosphotransferase or DIPP synthase; PPi-pyrophosphate; CMP, CDP, CTP- cytidine mono-, di-, tri- phosphate, respectively. The dashed red line represents the nucleophilic attack of the hydroxyl group (C3) of inositol-1-phosphate on the β-phosphoryl of CDP-inositol with formation of a phosphodiester bond. Figure 2: Catalytic reactions of IPCT/DIPPS bifunctional enzyme. Biosynthesis of di- myo -inositol-1,3′-phosphate-1′-phosphate (DIPP). IPCT-CTP:L- myo -inositol-1-phosphate cytidylyltransferase; DIPPS-CDP-L- myo -inositol: myo -inositolphosphotransferase or DIPP synthase; PPi-pyrophosphate; CMP, CDP, CTP- cytidine mono-, di-, tri- phosphate, respectively. The dashed red line represents the nucleophilic attack of the hydroxyl group (C3) of inositol-1-phosphate on the β-phosphoryl of CDP-inositol with formation of a phosphodiester bond. Full size image Here we present the three-dimensional structure of an archaeal CDP-alcohol phosphatidyltransferase (DIPPS) coupled with a cytidylyltransferase (IPCT) at 2.65 Å resolution. We analyse the functional role of highly conserved amino-acid residues by site-directed mutagenesis studies, dock substrates into identified pockets and propose a catalytic mechanism. This structure opens new avenues for homology modelling of other CDP-OH phosphotransferases, namely those with biomedical interest. Structure determination The bifunctional enzyme IPCT/DIPPS from A. fulgidus was produced in Escherichia coli and purified by immobilized metal affinity chromatography. The recombinant protein was crystallized from sample preparations using Triton X-100 for membrane extraction and protein solubilization. Crystals were grown using the in meso crystallization method [13] . They belong to the orthorhombic space group P2 1 2 1 2 with unit cell parameters of a =41.37, b =107.58 and c =123.95 Å ( Table 1 ). One IPCT/DIPPS molecule is present in the crystal asymmetric unit corresponding to a Matthews coefficient [14] of 2.87 Å 2 Da −1 and a solvent content of ~57%. This molecule interacts extensively with another molecule related by crystallographic symmetry ( Supplementary Fig. 1 ). The protein molecules are organized in the crystal as a stack of membrane layers, typical for in meso crystallization (type I membrane protein crystals [15] ), with interlayer contacts relying entirely on the IPCT cytoplasmic domain ( Supplementary Fig. 1 ). The structure was solved by molecular replacement using the coordinates of the IPCT domain we previously reported [16] and refined to a resolution of 2.65 Å with R work / R free values of 24.5% and 30%, respectively ( Table 1 ). The final model comprises 408 amino-acid residues, 1 magnesium ion, 9 water molecules and 4 lipid fragments. The electron density maps are generally of good quality ( Supplementary Fig. 2a ). The soluble IPCT domain is somewhat less ordered than the membrane DIPPS one (average B-factors of IPCT and DIPPS backbone atoms are 70.9 and 50.5 Å 2 , respectively; Supplementary Fig. 2b ). Table 1 Data collection and refinement statistics. Full size table Overall fold The IPCT/DIPPS bifunctional protein forms a dimer via its transmembrane (TM) domains ( Fig. 3a,b ). The dimeric interface is formed by helix TM4 of one protomer protruding between helices TM3′ and TM4′ of the other protomer and flanked by TM6. The interface is stabilized mostly by hydrophobic contacts within the lipidic bilayer and several H-bonds between polar/charged residues located at the cytoplasmic extramembrane side with a total contact area of 2,050 Å 2 . 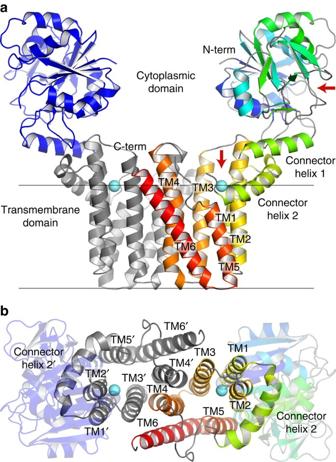Figure 3: X-ray structure of IPCT/DIPPS. The protein is dimerized via the TM domain. (a) One protomer is rainbow coloured and the other protomer (related by crystallographic symmetry) is in blue for cytoplasmic IPCT domain and grey for membrane DIPPS domain. Red arrows indicate the access to their active sites with a putative Mg2+drawn as a cyan sphere. Membrane surface position (grey) was calculated with PPM server49. (b) Top view of DIPPS domain (perpendicular to the membrane plane). Figure 3: X-ray structure of IPCT/DIPPS. The protein is dimerized via the TM domain. ( a ) One protomer is rainbow coloured and the other protomer (related by crystallographic symmetry) is in blue for cytoplasmic IPCT domain and grey for membrane DIPPS domain. Red arrows indicate the access to their active sites with a putative Mg 2+ drawn as a cyan sphere. Membrane surface position (grey) was calculated with PPM server [49] . ( b ) Top view of DIPPS domain (perpendicular to the membrane plane). Full size image DIPPS domain contains six TM α-helices TM1–TM6 and one shorter bent juxtamembrane helix (connector helix 2; Fig. 3a ). TM2 shows a kink around Asp357 nearby the membrane interface. The intracellular side of the TM domain is large and contains many polar and charged residues, whereas the opposite side is mostly embedded in the membrane. All TMs cross the membrane, except TM5, which is shorter. Connector helices 1 and 2 lie nearly parallel to the membrane plane, and link the soluble and membrane domains. We assigned connector helix 1 to IPCT and connector helix 2 to DIPPS, based on their distribution in the organisms where IPCT and DIPPS do not belong to the same polypeptide chain ( Supplementary Fig. 3 ). Although connector helix 2 is conserved among the DIPP-synthases, it is absent in many other CDP-alcohol phosphatidyltransferases ( Supplementary Fig. 4 ). It wraps around TM2 and the N terminus of TM5. Both connector helices are amphipathic, the hydrophobic side of connector helix 2 faces the membrane and is proximal to two lipid fragments, whereas its hydrophilic side point towards the cytoplasm and connector helix 1, whose apolar residues face the proximal β-sheet of IPCT. The cytoplasmic IPCT domain binds at the edge of the DIPPS domain ( Fig. 3a ). It comprises a core region formed by a central seven-stranded mixed β-sheet flanked by six α-helices. This arrangement is reminiscent of a dinucleotide-binding Rossmann fold, typical of nucleotidyltransferases, with an additional two-stranded β-sheet and a 30-residue long stretch. The sugar-binding region comprises a short antiparallel three-stranded β-sheet lying against the face of the central β-sheet where the nucleotide binds. The overall fold of the IPCT domain is very similar to the structure of that domain alone, which we previously reported [16] (root mean square deviation, r.m.s.d. of 0.6 Å for C α atoms). Interestingly, the IPCT domains dimerized in the crystals of the truncated one-domain construct [16] via the same interface that connects the IPCT and DIPPS domains in the full-length protein. Active site architecture and consensus sequence motif The six TM helices of DIPPS form a central hydrophilic cavity ~20 Å deep. This cavity is wide open (~10–20 Å) to the cytoplasm ( Fig. 3a ). Its entrance is flanked by three loops between TM2–TM3 (residues 369–373), connectors helix 1–helix 2 (residues 291–298), and TM4–TM5 (residues 430–440). The last two loops are less ordered suggesting flexibility ( Supplementary Fig. 2b ), and residues 292–294 and 430–433 were not included in the model as no electron density was visible in the maps. Remarkably, at one side of the cavity there are four aspartate residues (Asp357, Asp360, Asp378 and Asp382) pointing to the same patch of the electron density ( Fig. 4a ). The last three Asp are part of the conserved sequence pattern of CDP-alcohol phosphotransferase family, DG(x) 2 AR(x) 7,8 G(x) 3 D(x) 3 D, as defined in Prosite [17] , but all four aspartate residues are highlighted in the HMM logo of this family ( Fig. 4b ). Since Mg 2+ had been used throughout the purification of IPCT/DIPPS, we assigned a magnesium ion to this blob of density lying at the membrane interface. Mg 2+ is coordinated to the carbonyl of Asp357 and carboxylate groups of Asp357, Asp360 and Asp378 ( Fig. 4a ), where it is expected to decrease the pKa of the surrounding aspartate residues. Asp382 is not directly coordinated to the metal ion, but is within H-bonding distances to Asp357 and Asp378, and is ~4.5 Å away from Arg443. This cluster of negatively charged residues will tend to increase the pKa of neighbouring amino-acid residues. Because the coordination sphere of magnesium is still incomplete, it could also be engaged in binding of water molecules or the pyrophosphate moiety of CDP-inositol, as observed in some glycosyltransferases [18] and kinases [19] . 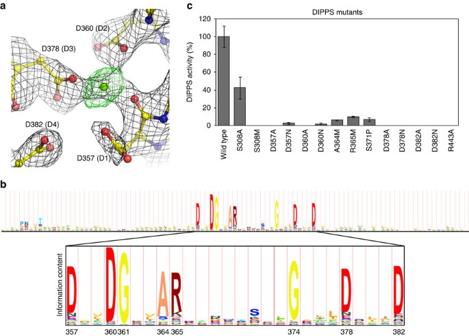Figure 4: DIPPS active site along with HMM logo and functional assays. (a) Zoomed view of the electron density map around the conserved aspartate residues. The maps were calculated before insertion of the magnesium ion in the model. The 2Fo–Fcdensity is shown in black and contoured at 1.5σ, the Fo–Fcdensity is green and contoured at 3σ; electron density around Asp357 is not very well defined. (b) HMM logo50around the consensus sequence of CDP-alcohol phosphotransferase family based on the alignment of 124 representative Pfam protein families as seeds51. The most conserved residues are located at the intracellular ends of TM2 and TM3. (c) Diagram of DIPPS activity as assessed in 30 min reactions to study the effect of point mutations; values are expressed as % relative to the wild type enzyme in the presence of 10 mM Mg2+. Values are averages of duplicate experiments derived from independent growths. Figure 4: DIPPS active site along with HMM logo and functional assays. ( a ) Zoomed view of the electron density map around the conserved aspartate residues. The maps were calculated before insertion of the magnesium ion in the model. The 2F o –F c density is shown in black and contoured at 1.5σ, the F o –F c density is green and contoured at 3σ; electron density around Asp357 is not very well defined. ( b ) HMM logo [50] around the consensus sequence of CDP-alcohol phosphotransferase family based on the alignment of 124 representative Pfam protein families as seeds [51] . The most conserved residues are located at the intracellular ends of TM2 and TM3. ( c ) Diagram of DIPPS activity as assessed in 30 min reactions to study the effect of point mutations; values are expressed as % relative to the wild type enzyme in the presence of 10 mM Mg 2+ . Values are averages of duplicate experiments derived from independent growths. Full size image Interestingly, the entries to the active sites of both enzymes that catalyse consecutive reactions in DIP synthesis are oriented in different directions ( Fig. 3a , red arrows). It is currently not known whether cross-talk exists between the two domains or if ipct/dipps gene fusion/separation produces any differences in the overall catalytic efficiency. It is possible that ligand binding could trigger rearrangements in the relative orientation of the two domains, as the interactions between IPCT and DIPPS domains are relatively weak (interface area of 479 Å 2 , solvation free-energy gain is −7.3 kcal mol −1 ; calculated with PISA [20] ). More studies are required to clarify these questions. Substrate binding sites and molecular docking While searching for potential substrate binding sites, we identified three pockets on the surface of DIPPS using HOLLOW [21] ( Fig. 5a ). Pocket 1 is the most interesting one, as it is flanked by the loop between TM2 and TM3, and lined by the family consensus residues Gly361, Ala364 and Gly374 ( Figs 5b and 6 ). Although IPCT/DIPPS protein was crystallized in the absence of substrates, residual 2F o –F c and F o –F c electron densities are seen in this region that cannot be accounted for by atoms of the protein. Pocket 2 is at the bottom of the hydrophilic cavity formed by strictly conserved residues among DIPPS proteins, namely Asn304, Arg305, Ser308, Ser354, Asp357 and Arg443 ( Fig. 6 ), sited on connector helix 2, TM2 and TM5. Pocket 3 is surrounded by helices TM4, TM5 and TM6, and loop TM5–TM6. Amino-acid residues from this loop are not conserved, and the pocket itself is far from the catalytic magnesium ion. Therefore, substrate binding within pocket 3 is very unlikely. Since pocket 1 comprises residues from the family consensus region ( Fig. 6 and Supplementary Fig. 4 ), it should be the binding site of the cytidine moiety, a common feature among substrates of all CDP-OH phosphotransferases. In contrast, pocket 2 includes connector helix 2 and its sequence conservation is restricted to enzymes assumed to have DIPP synthase activity, which suggests it to be the binding site of inositol-1-phosphate ( Fig. 5c ). 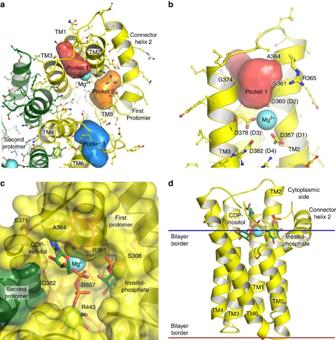Figure 5: Pockets visualization and substrate docking. (a) Putative ligand-binding pockets of DIPPS assigned with HOLLOW21(top view from the cytoplasm-facing side). The pockets are shown in pink (1), orange (2) and blue (3). (b) Detailed view of conserved pocket 1. The strictly conserved residues Gly361, Ala364 and Gly374, belonging to the family consensus sequence, form the surface of the pocket. (c) Model with bound ligands in DIPPS domain. The ligands fit well into the surface cavities and are properly oriented. (d) Position of DIPPS substrates relative to the bilayer surface. The CDP moiety is above the bilayer surface, whereas the inositol group of CDP-inositol and inositol-phosphate are slightly underneath it. The membrane position was estimated using the PPM server49. Figure 5: Pockets visualization and substrate docking. ( a ) Putative ligand-binding pockets of DIPPS assigned with HOLLOW [21] (top view from the cytoplasm-facing side). The pockets are shown in pink (1), orange (2) and blue (3). ( b ) Detailed view of conserved pocket 1. The strictly conserved residues Gly361, Ala364 and Gly374, belonging to the family consensus sequence, form the surface of the pocket. ( c ) Model with bound ligands in DIPPS domain. The ligands fit well into the surface cavities and are properly oriented. ( d ) Position of DIPPS substrates relative to the bilayer surface. The CDP moiety is above the bilayer surface, whereas the inositol group of CDP-inositol and inositol-phosphate are slightly underneath it. The membrane position was estimated using the PPM server [49] . 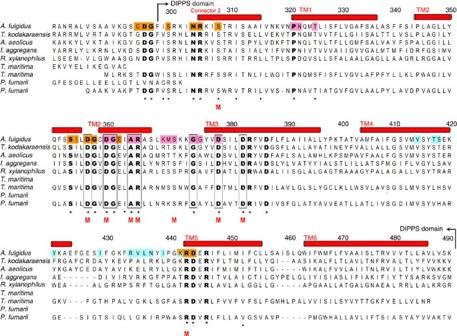Figure 6: Amino-acid sequence alignment of DIPP-synthases. Alignment was done with Geneious 6.0.3 ref.52based on DIPPS sequences from 33 organisms with confirmed or putative DIPP activity12. The selected sequences represent the major branches of phylogenetic tree12. Examples of products fromipct/dippsgenes fused (5) and separated (2).A., Archaeoglobus;T., Thermococcus;A.,Aquifex;I.,Ignisphaera;R.,Rubrobacter;T.,Thermotoga; andP.,Pyrolobus. Strictly conserved residues among all IPCT/DIPPS sequences are displayed in bold, and from the consensus pattern of CDP-alcohol phosphatidyltransferase family are enclosed in a box. Similar and identical residues are marked, respectively, with a dot and an asterisk beneath, and mutated residues by a red M. Residues involved in pocket formation are highlighted with pink (1), orange (2) and blue (3). Secondary structure elements represented with red tubes (α-helices) were assigned with DSSP53. Full size image Figure 6: Amino-acid sequence alignment of DIPP-synthases. Alignment was done with Geneious 6.0.3 ref. 52 based on DIPPS sequences from 33 organisms with confirmed or putative DIPP activity [12] . The selected sequences represent the major branches of phylogenetic tree [12] . Examples of products from ipct/dipps genes fused (5) and separated (2). A., Archaeoglobus ; T., Thermococcus ; A. , Aquifex ; I. , Ignisphaera ; R. , Rubrobacter ; T. , Thermotoga ; and P. , Pyrolobus . Strictly conserved residues among all IPCT/DIPPS sequences are displayed in bold, and from the consensus pattern of CDP-alcohol phosphatidyltransferase family are enclosed in a box. Similar and identical residues are marked, respectively, with a dot and an asterisk beneath, and mutated residues by a red M. Residues involved in pocket formation are highlighted with pink (1), orange (2) and blue (3). Secondary structure elements represented with red tubes (α-helices) were assigned with DSSP [53] . Full size image In order to find the best fit for the ligands within the proposed pockets, we used Autodock Vina software [22] for molecular docking. First, the smaller substrate, inositol-1-phosphate, was docked into pocket 2. Then, after inositol-1-phosphate was fixed in the best position, CDP-inositol docking simulations were run. The final CDP-inositol docked pose was chosen so that CMP moiety would reside inside the highly conserved region comprising, TM2, TM3 and loop TM2–TM3, with the phosphate groups close to the catalytic magnesium ion and the hydroxyl at C3 of inositol-1-phosphate. The best positions for the two docked substrates are displayed in Fig. 5c,d . Site-directed mutagenesis and functional assays The production of CDP-inositol and DIPP was quantified by 31 P-NMR in E. coli cell extracts ( Fig. 7 ). Divalent metal ions are known to be essential for the activity of CDP-OH phosphotransferases. IPCT/DIPPS is most efficient with Mg 2+ and no activity is observed without metal ions. 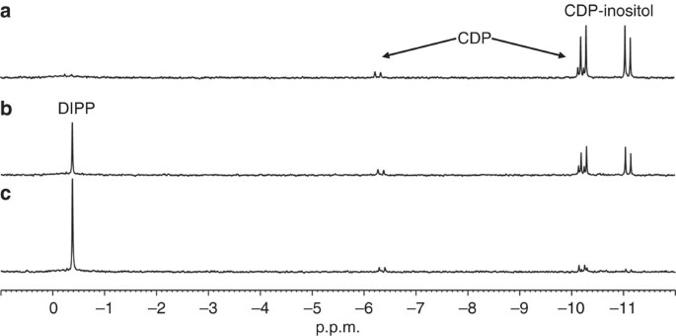Figure 7: Activity of the wild type IPCT/DIPPS and mutants assessed by31P-NMR. The nuclear magnetic resonance spectra show the production of CDP-inositol and DIPP resulting from 30 min incubation at 85 °C of reaction mixtures containing 2.7 mM of CTP, 7 mM of inositol-1-phosphate and cell extract ofE. coliproducingA. fulgidusIPCT/DIPPS (0.9 mg of total protein). (a) Point mutation S308M; (b) point mutation S308A; and (c) wild type. Spectra were acquired in a Bruker Avance II 500 spectrometer. Figure 7: Activity of the wild type IPCT/DIPPS and mutants assessed by 31 P-NMR. The nuclear magnetic resonance spectra show the production of CDP-inositol and DIPP resulting from 30 min incubation at 85 °C of reaction mixtures containing 2.7 mM of CTP, 7 mM of inositol-1-phosphate and cell extract of E. coli producing A. fulgidus IPCT/DIPPS (0.9 mg of total protein). ( a ) Point mutation S308M; ( b ) point mutation S308A; and ( c ) wild type. Spectra were acquired in a Bruker Avance II 500 spectrometer. Full size image Site-directed mutagenesis on conserved amino-acid residues from the family sequence pattern or considered functionally relevant (for example, for substrate binding) was carried out. HMM logo defines the conserved sequence of CDP-alcohol phosphotransferases as D1 357 (x) 2 D2 360 G 361 (x) 2 A 364 R 365 (x) 8 G 374 (x) 3 D3 378 (x) 3 D4 382 (superscript numbering corresponding to IPCT/DIPPS sequence; Fig. 4b ). Mutations of these aforementioned four aspartates to alanine or asparagine inactivated the enzyme, except for D357N, which resulted in a very low activity ( Fig. 4c ). These aspartate residues are part of the hydrophilic active site cavity and are close to the magnesium ion. Moreover, mutations of consensus residues Ala364 and Arg365 to methionine caused a considerable decrease of DIPPS activity ( Fig. 4c ). These residues are located at TM2 and lining pocket 1 ( Fig. 5b ). We speculate that A364M may obstruct the accessibility to the active site hydrophilic cavity, whereas R365M can affect the capture/binding of the negatively charged substrates. Mutation of equivalent residues (Ala to Gly and Arg to Ala) in Saccharomyces cerevisiae cholinephosphotransferase (CPT) also led to reduced catalytic activity, suggesting that both residues have a role in substrate binding or positioning [23] . Mutation of S371P within TM2–TM3 loop resulted in a significant reduction of the enzyme activity ( Fig. 4c ). This is probably owing to restraints on the loop flexibility that could affect the substrates entry. A similar result was also observed for the corresponding allele mutation in E. coli phosphatidylglycerophosphate synthase [24] . Related to pocket 2, we mutated Ser308, a strictly conserved amino-acid residue among enzymes with putative DIPPS activity, located on connector helix 2 that is adjacent to the inositol-1-phosphate binding pocket ( Figs 5c and 6 ). Decrease of DIPPS activity in S308A may be justified by the loss of H-bonding to the phosphate group of inositol-1-phosphate substrate, whereas enzymatic inactivation by S308M could result from introducing a bulkier side chain in the putative binding site, thus preventing substrate binding ( Fig. 4c ). Moreover, Arg443 sits at the bottom of the hydrophilic cavity and is within hydrogen bonding distances to Asp357 and Asp386 carboxylate groups, and one hydroxyl of the fitted inositol-1-phosphate and its substitution by alanine (R443A) abolishes DIPPS activity. The HMM logo sequence of CDP-OH phosphotransferases ( Fig. 4b ) compared with Prosite [17] reveals the conservation of an extra aspartate residue (D1, Asp357), which is not yet included in the consensus motif of this family. This Asp was also shown to be essential for the catalytic activity of other phosphotransferases [25] , likely having a role in substrate binding and positioning. We therefore propose to add this first aspartate residue in the consensus sequence pattern of CDP-OH phosphotransferases, as previously suggested [25] . Furthermore, some phosphatidylcholine synthases were shown to have 12 amino-acid residues between Arg and Gly [25] , so a more general conserved sequence pattern for CDP-alcohol phosphatidyltransferase family should be D (x) 2 DG(x) 2 AR(x) 7-12 G(x) 3 D(x) 3 D, to include all members of this family identified thus far (proposed changes highlighted in bold). Our site-directed mutagenesis studies on the consensus amino-acid residues ( Fig. 4b ) showed that all four aspartate, alanine and arginine residues are functionally relevant, as their loss abolishes or considerably reduces the catalytic activity ( Fig. 4c ). These results generally agree with data from the Sinorhizobium meliloti bacterial CPT [25] , S. cerevisiae CPT1 (ref. 23 ) and Brassica napus plant aminoalcoholphosphotransferase [26] (AAPT1), but the degree of reduction in their enzyme activities caused by the mutations may depend on the source and type of assays ( in vivo or in vitro ). A striking difference occurs when the second Asp (D2) is substituted by Ala; the small effect observed in yeast CPT1 and plant AAPT1 contrasts with the complete enzyme ablation of archaeal IPCT/DIPPS and bacterial CPT (also observed with D2N mutation). Indeed, this is the most conserved residue within CDP-OH_P_transf ( Fig. 4b ). These results imply that the eukaryotic CPT1 and AAPT1 should still be able to retain the divalent ion in the catalytic site of D2A mutants. Furthermore, no mutations were performed on the first Asp (D1) of yeast CPT1 and plant AAPT1, as it was not yet considered to be part of the family consensus motif. Notably, other family of peripheral membrane enzymes named phospholipase D, phosphatidylserine synthase type, which includes E. coli phosphatidylserine synthase, prokaryotic cardiolipin synthase, phospholipase D and some nucleases [23] shares a different motif (HxK(U) 4 D(x) 4 UUGO). These enzymes catalyse the transfer of a substituted phosphate group, other than diphosphate or nucleotidyl residues, from one compound (donor) to another (acceptor). Although they appear capable of forming an identical phosphoester bond [27] , [28] they do not require a divalent ion for catalysis and follow a ping-pong reaction type with an enzyme-bound intermediate [29] , [30] , [31] . In contrast, kinetics studies on members of CDP-alcohol phosphotransferase family, such as synthases of phosphatidylserine from yeast [29] , [32] and Bacillus licheniformis [33] , phosphatidylglycerophosphate from E. coli [34] and phosphatidylcholine from rat [35] , suggest a sequential Bi–Bi mechanism for these enzymes. Assuming also a single displacement S N 2-like mechanism for DIPPS, we propose that Asp357/Asp382 function as base catalysts and promote the direct nucleophilic attack of the hydroxyl group (on C3) of inositol-1-phosphate on the β-phosphoryl of CDP-inositol with formation of DIPP and CMP ( Fig. 2 ). Remarkably, the membrane character of DIPP synthase is intriguing, as all its substrates and products are water soluble ( Fig. 2 ). A recent evolution analysis of DIPP-synthases has shown that these enzymes evolved from phosphatidylinositol synthases that are membrane proteins, so DIPPS kept the membrane-spanning character of its ancestor [12] . In contrast, CDP-OH_P_trans enzymes involved in phospholipid biosynthesis usually have a lipophilic substrate that can either be a donor substituent or alcohol acceptor (for example, diacylglycerol (DAG)) that reacts with a water-soluble one (typically a phospholipid head group, for example, glycerol or serine). However, some enzymes, such as cardiolipin synthases, have two lipidic substrates, CDP-DAG and phosphatidylglycerol. The X-ray structure of IPCT/DIPPS revealed a large polar active site cavity that lies near the membrane interface and should be a common feature to other CDP-OH phosphotransferases. This positioning is strategic to allow accommodation and binding of both hydrophilic and lipophilic substrates. The catalytic reaction occurs at the hydrophilic–hydrophobic interface of the membrane with Mg 2+ lying on the border ( Fig. 5d ), so the lipophilic chains of diacylglycerol or other phospholipids could easily be embedded in the lipid bilayer. We expect a high degree of structural conservation among CDP-alcohol phosphotransferases around the consensus region, located at the N terminus of their sequences (TM2–TM3 in DIPPS) with subtle or more significant differences on the ligand-binding sites depending on their substrates. Members of this family are involved in the synthesis of phospholipids, which have important roles in cell viability and infectivity of pathogenic bacteria [1] , [2] , [4] , [36] . Therefore, DIPPS structure may be of utmost value to structural homology modelling and in providing molecular targets for the rational design of novel drugs. Expression and purification The A. fulgidus AF0263 gene encoding IPCT/DIPPS was amplified by PCR (forward primer: 5′-TCCC CCCGGG ATGATAAATGTTGACGGAGAATAC-3′, Xma I site underlined; reverse primer: 5′-GCG GAGCTC TTTAGAAACCAAAACAGCAAGTAAAG-3′, Sac I site underlined). The PCR product was cloned into the expression vector pET52b(+) (Novagen) using Sac I and Xma I restriction sites, with N-terminal Strep tag II and C-terminal His 10 tag. The resulting plasmid was verified by DNA sequencing. The expression vector was transformed into E. coli C43 DE3. Cells were cultivated in terrific broth medium at 37 °C in a 30-litre fermentor with pH controlled at 7.4, and induced with 0.5 mM isopropyl β-D-1-thiogalactopyranoside when the OD 600 reached 1.0. The temperature was subsequently lowered to 30 °C. Cells were harvested 6 h following induction and resuspended in lysis buffer (50 mM sodium citrate, 50 mM sodium phosphate, 200 mM NaCl, 5% glycerol, 100 mM sucrose, 1 mM ethylenediaminetetraacetic acid, 0.5 mM phenylmethanesulfonylfluoride, 2 mM β-mercaptoethanol and protease inhibitors cocktail tablet SIGMAFAST; pH 7.5). Cells were disrupted using a constant flow cell disruptor, and cell debris and inclusion bodies were removed by centrifugation at 10,000 g for 30 min. E. coli membranes were isolated by ultracentrifugation at 200,000 g for 2 h. The protein was extracted from the membranes by solubilization in 2% Triton X-100, 20% glycerol, 1 M NaCl, 50 mM phosphate buffer, 50 mM imidazole, 100 mM sucrose, 2 mM β-mercaptoethanol and 1 mM MgCl 2 (final pH 7.4 at 277 K) for 2 h. Insoluble fraction was separated by 1 h centrifugation at 100,000 g . The supernatant was loaded onto HisTrap HP column (GE Healthcare). The loaded sample was washed with buffer A (0.1% Triton X-100, 50 mM phosphate buffer, 50 mM imidazole, 10% glycerol and 1 M NaCl; pH 7.4), followed by an additional wash with buffer A supplemented with 110 mM imidazole. The protein was eluted with buffer B containing 0.1% Triton X-100, 50 mM phosphate buffer, 500 mM imidazole, 10% glycerol, 300 mM NaCl and 1 mM MgCl 2 ; pH 7.4. Immediately after elution, the sample was supplemented with 1 mM β-mercaptoethanol and concentrated to ~20 mg ml −1 in centrifugal filter unit with a membrane of 100 kDa molecular weight cutoff. Biochemical characterization of IPCT/DIPPS Point mutations were introduced using QuickChange I kit (Agilent Technologies) and confirmed by DNA sequencing (STAB VIDA). Primers designed for the mutants are listed in Supplementary Table 1 . The mutants were cultured following a similar protocol as described for the wild type. SDS-PAGE and His-tag western blotting were performed on the membrane preparations from cell extracts, confirming that all mutants were expressed in the E. coli membranes ( Supplementary Fig. 5a,b ). Protein content was estimated by the Bradford method [37] . Inositol-1-phosphate was produced from glucose-6-phosphate by the activity of A. fulgidus inositol-1-phosphate synthase, and purified by ion exchange chromatography (QAE-Sephadex A-25 and Dowex 50W-X8 resins) [8] . The IPCT/DIPPS activities were assessed in cell extracts of E. coli C43, harbouring wild type or mutant variants of the ipct / dipps gene from A. fulgidus . The cell pellets were suspended in 50 mM Bis/Tris/propane-HCl (pH 8.0) containing 5% (v/v) glycerol and 100 mM NaCl; cells were disrupted in a French press and debris were removed by centrifugation (10,000 g , 15 min, 4 °C). Reaction mixtures (0.3 ml) containing 25 mM Bis/Tris/propane-HCl (pH 8.0), 10 mM MgCl 2 , 2.7 mM CTP and 7 mM inositol-1-phosphate, and cell extract (0.9 mg of total protein) were incubated at 85 °C for 1 and 30 min. The reactions were stopped on ice before the addition of deuterated water (200 μl) and 25 mM EDTA (pH 8.0). The reaction products of IPCT and DIPPS, that is, CDP-inositol and DIPP, respectively, were quantified by 31 P-NMR using diglycerol-phosphate as an internal concentration standard ( Fig. 7 ). Owing to the bifunctionality of IPCT/DIPPS, the IPCT activity served also as a reliable control for protein production. The concentration of the IPCT product was fairly constant for the 14 mutants examined ( Supplementary Fig. 5b ). All these assays were performed in duplicate corresponding to independent growths. Crystallization and structure determination The crystals of IPCT/DIPPS were grown using an in meso crystallization method [13] , similarly to Gordeliy et al. [38] The protein–mesophase mixture contained concentrated enzyme solution and monoolein. High-throughput crystallization was performed with NT8 robot (Formulatrix, USA). Plate-like crystals reaching the size of 5 × 20 × 200 μm were grown in 50 nl protein-containing mesophase drops overlaid by precipitant solution (4–12% PEG 550–6,000, 0.2–2 M sodium malonate, pH 5.8–8.2) at 295 K for 30–300 days. The crystals were harvested directly from the mesophase matrix and flash-frozen in liquid nitrogen. The best X-ray diffraction data were collected from two crystals at 100 K, 0.8726 Å wavelength, on ID23-1 and ID23-2 beamlines of the European Synchrotron Radiation Facility (Grenoble, France). Data of these two crystals were merged and integrated to 2.65 Å ( R pim in the highest resolution shell is 46.9% with CC of 51.3% and I/σI of 1.7; Table 1 ), according to Karplus and Diederichs [39] , with MOSFLM [40] and scaled using Scala [41] from CCP4 software suite [42] . Initial phases were obtained via Molecular Replacement with MOLREP [43] using the crystallographic structure of the soluble domain (PDB ID 2XME) as a starting model. The electron density maps revealed that the soluble domains form layers with a separation of ~70 Å that is enough for the membrane-like layer containing TM domains. Additional search for alpha-helical fragments resulted in establishment of position of five TM alpha-helices. Refinement of the fragments’ structure with Refmac5 (ref. 44 ) and PHENIX [45] resulted in improvement of the electron density maps, and following identification of the sixth TM helix and two alpha-helices parallel to the membrane plane. Eventually, identities of the side chains were determined. The final R-factors are 24.3 and 30.0% ( R and R free , respectively). Ramachandran plot shows that 96.3% of the amino-acid residues are in favoured regions, 3.2% are in allowed regions and 0.5% in not allowed regions. All structural figures were prepared with CCP4mg [46] and PyMOL [47] . Molecular docking studies Autodock Vina software [22] was used for molecular docking along with Autodock/Vina plugin for PyMOL to set up the simulations. Autodock Vina uses as default the Iterated Local Search global optimization algorithm for an efficient global search. For the local optimization, Autodock Vina uses a quasi-Newton, Broyden–Fletcher–Goldfarb–Shanno method. The docking was performed within the axis-aligned bounding box in the cytoplasmic part of the TM domain that contains all three binding pockets visualized using HOLLOW [21] ( Fig. 5a–d ). The volume of the search space was ~20,000 A 3 . During the docking, ligands were flexible, that is, all non-aromatic bonds were rotatable. The magnesium ion was included in the calculations. First, the smaller compound inositol-1-phosphate was docked around pocket 2. During this simulation, four amino-acid residues flanking the binding pocket, Asp296, Ser300, Arg305 and Arg365, were allowed to change their conformations. Then, after inositol-1-phosphate was fixed in the best position, CMP docking simulations were run with a single flexible residue, Arg365. The scoring function used by Autodock Vina is given as a weighted sum of steric interactions, hydrophobic interactions and, where applicable, hydrogen bonding [22] . Because this software energy (scoring) function, similarly to others used in computational docking, is usually not enough to discriminate the correct docking pose from other poses [48] , the 100 top-ranking possible ligand positions were generated by the Vina software, and the best one was chosen according to the biochemical rationales. Accession codes : Coordinates and structure factors have been deposited in the Protein Data Bank with accession code 4MND . How to cite this article: Nogly, P. et al. X-ray structure of a CDP-alcohol phosphatidyltransferase membrane enzyme and insights into its catalytic mechanism. Nat. Commun. 5:4169 doi: 10.1038/ncomms5169 (2014).